2′-OMe-phosphorodithioate-modified siRNAs show increased loading into the RISC complex and enhanced anti-tumour activity Improving small interfering RNA (siRNA) efficacy in target cell populations remains a challenge to its clinical implementation. Here, we report a chemical modification, consisting of phosphorodithioate (PS2) and 2′- O -Methyl (2′-OMe) MePS2 on one nucleotide that significantly enhances potency and resistance to degradation for various siRNAs. We find enhanced potency stems from an unforeseen increase in siRNA loading to the RNA-induced silencing complex, likely due to the unique interaction mediated by 2′-OMe and PS2. We demonstrate the therapeutic utility of MePS2 siRNAs in chemoresistant ovarian cancer mouse models via targeting GRAM domain containing 1B (GRAMD1B), a protein involved in chemoresistance. GRAMD1B silencing is achieved in tumours following MePS2-modified siRNA treatment, leading to a synergistic anti-tumour effect in combination with paclitaxel. Given the previously limited success in enhancing siRNA potency with chemically modified siRNAs, our findings represent an important advance in siRNA design with the potential for application in numerous cancer types. Small interfering RNA (SiRNA)-based therapies have shown promise in recent clinical trials as anti-cancer agents [1] , [2] . This technology offers tremendous potential in silencing ‘non-druggable’ targets that are not amenable to conventional therapeutics such as small molecules or monoclonal antibodies [3] , [4] . However, the lack of stability and low potency at target sites following systemic administration remain the major obstacles to clinical translation of this therapy [5] , [6] . To overcome these problems, efforts have been made to chemically modify the 2′-position of the ribose moiety (for example, 2′-OMe or 2′-F) or phosphate backbone of the siRNA molecule (for example, phosphoromonothioate (PS) modification) such that enhanced serum stability [7] , bioavailability [8] and prolonged duration of action [9] could be achieved (Reviewed in ref. 10 ). Importantly, combining PS and 2′-modification impart superior stability over single modifications [11] , [12] , leading to the approval of Kynamro, an antisense therapeutic, by the Food and Drug Administration [13] . Despite the advance, combination of PS and 2′-modification shows limited enhancement of siRNA potency [14] . Moreover, synthesis of PS or MePS by standard phosphoramidite methodology also generates a mixture of unresolvable diastereomeric oligomers, which could potentially result in variable biochemical, biophysical and biological properties. We have recently reported that PS2 modification, which substitutes sulphur atoms for both of the non-bridging phosphate and oxygen atoms, significantly improves serum stability and gene silencing over PS-modified siRNAs [15] . Its achiral nature at the phosphorous centre eliminates the generation of isomeric by-products, thereby permitting batch–to-batch quality control [16] , [17] , a feature that cannot be achieved with the MePS platform. As such, PS2-modified siRNA is a prime candidate for introducing critical new features to further improve siRNA efficacy both in vitro and in vivo . We hypothesized that the incorporation of two most widely used sugar modifications, 2′-OMe or 2′-F, into a PS2-modified construct could lead to further enhancement of the PS2 siRNA stability and increase their clinical potential. In this study, we show that the novel MePS2 design significantly enhances serum stability and silencing activity of siRNAs. This enhanced potency stems from an unforeseen increase in the loading of siRNAs to the RNA-induced silencing complex (RISC). We further demonstrate the therapeutic utility of MePS2-modified siRNAs by targeting GRAM domain containing 1B (GRAMD1B), a novel gene identified through a whole-genome, taxane sensitivity screen. Given that limited success has been achieved thus far towards broadly enhancing siRNA potency with chemically modified siRNAs [18] , [19] , [20] , MePS2 modification represents a major new direction for enhancing the clinical application of existing RNA interference (RNAi)-based therapies. Synthesis and activity of chemically modified siRNAs To investigate the gene-silencing activity of MePS2– or FPS2–siRNAs and to gain insight into their regulation of the RNAi pathway, we first synthesized these novel siRNAs via the solid-phase synthesis technique. Given our extensive experience in using unmodified (UM) siRNAs to target EPH receptor A2 (EphA2), a tyrosine kinase receptor that promotes tumour progression in cancer [21] , we chose to initially evaluate our novel siRNAs using EphA2 as a model system. We have previously identified favourable positions of PS2 modification using a siRNA that targets green fluorescence protein ( Supplementary Fig. 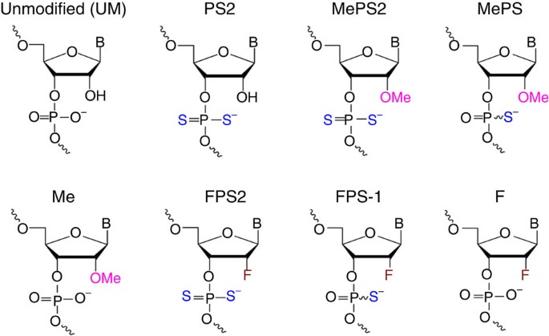Figure 1: Chemical structures of modified siRNAs. Chemical structures of modified siRNAs used for the initial screen. 1 ; Supplementary Table 1 ). The silencing efficacy of selected PS2-modified sequences was further validated using another siRNA sequence [15] . Informed by these prior observations, we designed MePS2/FPS2-1 through -3 constructs for siEphA2 ( Fig. 1 , Table 1 ). We also created MePS2/FPS2-4 sequences, where there are two MePS2/FPS2 groups present at the seed region of the antisense strand. Finally, counterpart sequences were synthesized with either 2′-OMe/2′-F alone, PS2 alone or MePS/FPS placed at the same locations. Figure 1: Chemical structures of modified siRNAs. Chemical structures of modified siRNAs used for the initial screen. Full size image Table 1 Chemical structures of modified siRNAs. Full size table SKOV3ip1 and HeyA8, both epithelial ovarian cancer (OvCa) cell lines that highly express EphA2, were transfected with synthesized siRNAs in serum-free conditions to test silencing efficacy. Two independent experiments were performed and EphA2 protein quantification was done at 48 h post transfection. MePS2-1, MePS2-2, Me-4, FPS-1, FPS-4 and F-1 significantly decreased EphA2 levels in SKOV3ip1 compared with UM siRNA and outperformed their counterparts ( Fig. 2a ). In particular, we found that the MePS2-1 modification silenced EphA2 to a much greater degree compared with UM (sixfold enhancement). It also showed 4, 7.5 and 7-fold enhancement in EphA2 silencing compared with PS2-1-, MePS-1- and Me-1-modified sequences, respectively. In contrast to MePS2-1 and MePS2-2, FPS2-1 and FPS2-2 modifications did not increase silencing efficiency of the siRNA. Given the significant improvement in gene silencing observed with MePS2-1, we focused our subsequent effort on Me-modified constructs. In HeyA8 cells, MePS2-1-modified siEphA2 also showed superior silencing activity compared with the UM sequence (80% versus 50% knockdown, respectively, Fig. 2b ). Interestingly, both PS2-1- and PS2-2-modified sequences resulted in significant silencing of EphA2 in this cell line. 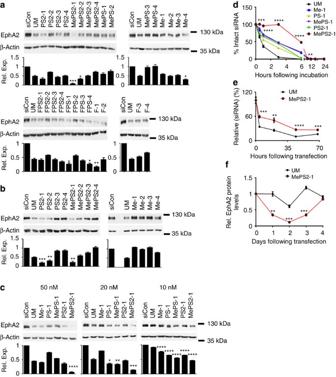Figure 2: Stability and gene-silencing activity of chemically modified siRNA. (a) Knockdown of EphA2 in SKOV3ip1 cells using chemically modified siRNAs (100 nM, serum-free condition). (b) Knockdown of EphA2 using selected siRNA sequences in HeyA8 cells (100 nM, serum-free condition). (c) Knockdown of EphA2 using chemically modified siRNAs in SKOV3ip1 cells (10, 20 and 50 nM, 10% FBS-containing media). (a–c) Cells were treated with siRNAs for 4 h and EphA2 protein levels were examined 48 h post transfection. (d) Stability of chemically modified siRNAs in 10% FBS at 37 °C. (e) Intracellular stability of UM and MePS2-1-modified siEphA2 in SKOV3ip1 cells (50 nM, serum-free condition). (f) Duration of EphA2 knockdown following UM and MePS2-1-modified siEphA2 treatment in SKOV3ip1 cells (50 nM, 10% FBS-containing media). (P-values obtained with Student’st-test; *P<0.05; **P<0.01; ***P<0.001; or ****P<0.0001; compared with UM siEphA2 sequence; bars and error bars represent mean values and the corresponding s.e.m.s (n=3).) Figure 2: Stability and gene-silencing activity of chemically modified siRNA. ( a ) Knockdown of EphA2 in SKOV3ip1 cells using chemically modified siRNAs (100 nM, serum-free condition). ( b ) Knockdown of EphA2 using selected siRNA sequences in HeyA8 cells (100 nM, serum-free condition). ( c ) Knockdown of EphA2 using chemically modified siRNAs in SKOV3ip1 cells (10, 20 and 50 nM, 10% FBS-containing media). ( a – c ) Cells were treated with siRNAs for 4 h and EphA2 protein levels were examined 48 h post transfection. ( d ) Stability of chemically modified siRNAs in 10% FBS at 37 °C. ( e ) Intracellular stability of UM and MePS2-1-modified siEphA2 in SKOV3ip1 cells (50 nM, serum-free condition). ( f ) Duration of EphA2 knockdown following UM and MePS2-1-modified siEphA2 treatment in SKOV3ip1 cells (50 nM, 10% FBS-containing media). ( P -values obtained with Student’s t -test; * P <0.05; ** P <0.01; *** P <0.001; or **** P <0.0001; compared with UM siEphA2 sequence; bars and error bars represent mean values and the corresponding s.e.m.s ( n =3).) Full size image Given the promise of the MePS2-1 modification in both of the cell lines examined, we next investigated the impact of different modifications at the same position on gene silencing and serum stability ( Supplementary Fig. 2 ; Fig. 2c,d ). To mimic the condition in the preclinical or clinical setting, sequences were introduced into SKOV3ip1 cells in media containing 10% fetal bovine serum (FBS). EphA2 protein levels were examined 48 h post transfection. MePS2-1 displayed a significant improvement over all other sequences tested, including PS2-1 ( Fig. 2c ; Supplementary Fig. 3 ). Of note, further modifications at different positions of the MePS2-1 siEphA2 sequence resulted in reduced silencing efficiency ( Supplementary Fig. 4 ). The improved gene silencing as the result of MePS2-1 modification was also observed when another siRNA sequence was used (parathymosin-targeted siRNA, Supplementary Fig. 5a ). SiRNA stability assays show that the majority of UM siRNA was broken down within 20 min, with near-complete degradation at 3 h ( Fig. 2d ). Overall improvements in serum stability were seen for all modified sequences in comparison to UM, but MePS2-1 displayed the highest sequence stability, with a large portion of the input molecules remaining intact at 3 h. An even greater enhancement in stability was observed with parathymosin-targeted siRNA ( Supplementary Fig. 5b ). We next wondered if the enhanced stability after modification accounted for these constructs’ increased silencing efficacy. To test this, we employed stemloop polymerase chain reaction (PCR) technique to quantify intact siRNA within the cell following transfection ( Fig. 2e ; Supplementary Fig. 5c ). Increased intracellular siRNA stability via MePS2 modification was confirmed, but not to a degree that would explain its dramatic increase in siRNA potency. Our conclusion was that MePS2-1 showed increased potency independent of improvements in stability. This was consistent with the finding that the duration of silencing was not significantly prolonged for MePS2-1 sequence compared with the UM counterpart ( Fig. 2f ). Biophysical properties of MePS2-1 siRNA We examined the mechanism by which MePS2-1 sequence enhances the gene-silencing effect. First, we examined thermodynamic stability (measured by RNA duplex melting temperature ( Tm) ) since the destabilization of the 5′-end of duplex by introducing modified units into 3′-end of the sense strand is crucial in creating favourable thermodynamic asymmetry for siRNA activity [15] , [22] , [23] . Measuring the Tm of MePS2-1 and its counterpart sequences showed MePS2-1 to have the largest decrease in Tm (1.24 °C, Δ Tm , P <0.05) when compared with UM siRNA, suggesting duplex unwinding may have a role in its enhanced RNAi activity ( Table 2 ). Importantly, in contrast to 2′-OMe modification alone which increased T m, its addition at the site of PS2 modification did not elevate Tm . Table 2 Thermostability of chemically modified siRNAs. Full size table We also hypothesized that the MePS2 modification may potentially alter helix conformation between the target and guide strand by changing local structure, which can affect silencing activity [24] , [25] . However, circular dichroism (CD) spectra of all the modified sequences tested were similar to the spectrum of UM duplexes and are consistent with the typical A-type structure (a maximum of the positive Cotton effect at 268 nm and a crossover point at 240 nm) ( Fig. 3a ). 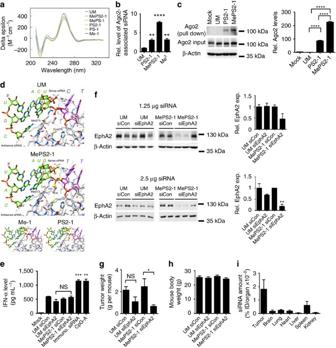Figure 3: Biophysical properties of MePS2-1 siRNA. (a) CD spectra of Me-1, PS-1, MePS-1, PS2-1 and MePS2-1-modified siEphA2s. (b) Intracellular binding of UM, PS2-1, MePS2-1 and Me2modified siEphA2 to Ago2 protein in SKOV3ip1 cells (50 nM, serum-free condition). (c) Ago2 association with UM, PS2-1 and MePS2-1 biotin-labelled siRNAs. Apart from mock-treated (no treatment control) sample, each sample contains the same amount of siRNA (quantified using stemloop PCR). Transfection was performed using 50 nM biotin-labelled siRNA in serum-free condition. The bottom two panels show the effect of transfection on total Ago2 level in cells. (d) Computational modelling of the siRNA:PAZ interaction. UM, MePS2-1, Me-1 and PS2-1-modified siRNAs were modelled, all shown in the same orientation. (e) Induction of IFN-α by UM and MePS2-1-modified siEphA2 in C57BL/6-derived dendritic cells (75 nM, serum-free condition). A high IFN-α-inducing siRNA sequence and CpG2216were used as positive controls. (f) Knockdown of EphA2 protein in tumours following a single dose of siRNA-DOPC treatment in SKOV3ip1 OvCa mouse model (1.25 and 2.5 μg per dose). Effect of UM-siEphA2-DOPC and MePS2-1-siEphA2-DOPC on tumour burden (g) and body weight (h) in SKOV3ip1 orthotopic OvCa mouse model following 4 weeks of siRNA treatment (n=10). (i) Biodistribution of MePS2-1-siEphA2-DOPC. SiRNA levels were measured in various organs at 24 h post i.p. administration. Stemloop PCR technique was employed to assess intact siRNA levels. The total amount of siRNA in each organ was measured (n=4) and was expressed as percentage of injected dose (ID). (P-values obtained with Student’st-test; (b) **P<0.01; ****P<0.0001; compared with UM; (c) ****P<0.0001; compared with respective controls; (e) **P<0.01; ***P<0.001; compared with UM siCon; (f,g) *P<0.05 or **P<0.01; compared with the corresponding control groups; bars and error bars represent mean values and the corresponding s.e.m.s (n=2–3).) Figure 3: Biophysical properties of MePS2-1 siRNA. ( a ) CD spectra of Me-1, PS-1, MePS-1, PS2-1 and MePS2-1-modified siEphA2s. ( b ) Intracellular binding of UM, PS2-1, MePS2-1 and Me 2 modified siEphA2 to Ago2 protein in SKOV3ip1 cells (50 nM, serum-free condition). ( c ) Ago2 association with UM, PS2-1 and MePS2-1 biotin-labelled siRNAs. Apart from mock-treated (no treatment control) sample, each sample contains the same amount of siRNA (quantified using stemloop PCR). Transfection was performed using 50 nM biotin-labelled siRNA in serum-free condition. The bottom two panels show the effect of transfection on total Ago2 level in cells. ( d ) Computational modelling of the siRNA:PAZ interaction. UM, MePS2-1, Me-1 and PS2-1-modified siRNAs were modelled, all shown in the same orientation. ( e ) Induction of IFN-α by UM and MePS2-1-modified siEphA2 in C57BL/6-derived dendritic cells (75 nM, serum-free condition). A high IFN-α-inducing siRNA sequence and CpG 2216 were used as positive controls. ( f ) Knockdown of EphA2 protein in tumours following a single dose of siRNA-DOPC treatment in SKOV3ip1 OvCa mouse model (1.25 and 2.5 μg per dose). Effect of UM-siEphA2-DOPC and MePS2-1-siEphA2-DOPC on tumour burden ( g ) and body weight ( h ) in SKOV3ip1 orthotopic OvCa mouse model following 4 weeks of siRNA treatment ( n =10). ( i ) Biodistribution of MePS2-1-siEphA2-DOPC. SiRNA levels were measured in various organs at 24 h post i.p. administration. Stemloop PCR technique was employed to assess intact siRNA levels. The total amount of siRNA in each organ was measured ( n =4) and was expressed as percentage of injected dose (ID). ( P -values obtained with Student’s t -test; ( b ) ** P <0.01; **** P <0.0001; compared with UM; ( c ) **** P <0.0001; compared with respective controls; ( e ) ** P <0.01; *** P <0.001; compared with UM siCon; ( f , g ) * P <0.05 or ** P <0.01; compared with the corresponding control groups; bars and error bars represent mean values and the corresponding s.e.m.s ( n =2–3).) Full size image Our next hypothesis was that the thiol groups on MePS2-1’s phosphate backbone may interact with metal ions or amino-acid residues in RISC to increase the sequence’s affinity for the complex [26] , [27] . We tested this hypothesis by transfecting UM, PS2-1 and MePS2-1 into SKOV3ip1 cells, then immunoprecipitating argonaute-2 (Ago2). SiEphA2 with two 2′-OMe residues at the 5′-end of the sense strand (Me 2 -siEphA2) [28] was used as a positive control. From a panel of 10 different microRNAs (miRNA) tested, hsa-miR-484 was found to be both unaffected by siEphA2 and present at a high level in SKOV3ip1 cells, thus we chose it as our normalizing control ( Supplementary Fig. 6 ). We found that Ago2-associated MePS2-1 and PS2-1 sequences were enriched sevenfold and threefold compared with UM siRNA, respectively ( Fig. 3b ). In contrast to UM siRNA where the level of associated Ago2 protein was below the limit of detection via western blotting, a high level of siRNA-associated Ago2 was detected for both PS2-1 and MePS2-1 siRNAs in the biotin-siRNA pull-down study ( Fig. 3c ). In both of these experiments, there was a significant increase in Ago2 binding for MePS2-1 compared with PS2-1 sequence (greater than twofold). The ability of MePS2-1 modification to enhance loading of siRNAs into RISC was also demonstrated using another siRNA sequence ( Supplementary Fig. 5d ). Of note, the enhanced binding of MePS2-1 siRNAs to RISC had minimal effect on miR biogenesis ( Supplementary Fig. 7 ). We further investigated the impact of MePS2-1 modification on strand loading. SKOV3ip1 cells were transfected with siEphA2 sense (S) and antisense (AS) strand-specific luciferase reporters. MePS2-1(S) decreased the luciferase signal to a much greater degree (2.2-fold enhancement) compared with UM siRNA in cells transfected with the AS reporter construct ( Supplementary Fig. 8a ). As expected, MePS2-1(AS) did not reduce the luciferase signal significantly when compared with control siRNA (siCon) treatment. Conversely, in cells transfected with the S reporter construct, MePS2-1(AS) further improved the silencing ability of the siRNAs when compared with the UM sequence, while no silencing was observed with MePS2-1(S) ( Supplementary Fig. 8b ). We further compared the silencing efficacy of MePS2-1(S) with Me 2 (S)-siRNA. In cells transfected with the AS reporter construct, Me 2 (S) siRNAs decreased the luciferase signal to a greater extent compared with UM, as expected ( Supplementary Fig. 8a ). This extent of silencing was comparable with that achieved by MePS2-1(S). The addition of MePS2-1(S) modification to Me 2 (S)-siRNA (Me 2 MePS2-1) did not significantly alter its silencing efficiency. These results are consistent with the level of EphA2 mRNA knockdown observed with these siRNAs ( Supplementary Fig. 8c ). We used computational modelling to examine the potential effects of the MePS2 modification on the interaction of siRNAs with RIC, focusing on the PAZ domain that recognizes 3′-overhanging nucleotides of siRNA duplexes [29] . In the crystal structure, the siRNA 5′-(CGUGACU)-d(CU)-3′ forms a duplex with one G-G and two U-C mismatch pairs and 3′-terminal d(CU) overhangs. Modelling entailed changing the penultimate 3′-dC to T, converting the terminal RNA U-C pair in the native duplex to G:C, and changing the adjacent G:C pair to A:U. Methyl groups were also added to the sugar 2′-oxygen atoms of U and G in the antiperiplanar orientation (torsion angle C3′-C2′-O2′-C methyl (ref. 30 )). Inspection of the model of MePS2-1 bound to PAZ indicates that the combination of the 2′-OMe and PS2 modifications will likely benefit the interaction between siRNA and PAZ ( Fig. 3d ). Thus, the proximities of the 2′-OMe moiety of G and Cε of M273 as well as the PS2 moiety of T and both Cε of Met273 and the sulfhydryl group of C270 are consistent with favourable hydrophobic interactions that are absent in the complex with the UM siRNA and are superior to those for the Me-1 and PS2-1 siRNAs. Taken together, the combination of PS2 and 2′-OMe modification triggers an unusual stereoelectronic effect in the backbone of the siRNA, which leads to increased RISC loading. This, along with an increase in resistance to nuclease degradation as well as a decrease in Tm , provides a likely explanation for enhanced RNAi activity by MePS2-1 modification. In vivo application of MePS2-1 siRNA Having identified a promising chemical modification that could significantly enhance the stability and silencing activity of siRNAs, we next characterized its potential off-target immunotoxicity. C57BL/6-derived dendritic cells were treated with UM siCon, UM siEphA2, MePS2-1 siCon and MePS2-1 siEphA2. Interferon alpha (IFN-α) levels, a surrogate marker for non-specific induction of innate immunity, were similar for all four sequences examined ( Fig. 3e ). No difference in Toll-like receptor 7 (TLR7)-induced IFN-α or tumour necrosis factor alpha (TNF-α) levels was observed between UM siEphA2 and MePS2-1 siEphA2 at all time points examined ( Supplementary Fig. 9 ). Of note, serum IFN-α and TNF-α levels were both undetectable at 2, 6 and 24 h following intraperitoneal (i.p.) administration of 1,2-dioleoyl-sn-glycero-3-phosphatidylcholine (DOPC) nanoliposomes-delivered UM-siEphA2 (UM-siEphA2-DOPC) or MePS2-1 siEphA2 (MePS2-1-siEphA2-DOPC) in mice. The efficacy of the MePS2-1 siRNA in vivo was next assessed using an orthotopic mouse model of OvCa (SKOV3ip1). The effect of EphA2 knockdown in tumours was first examined following a single injection. While some degree of knockdown was achieved with MePS2-1-siEphA2-DOPC at the dose of 1.25 μg, ( Fig. 3f ), >2.5 μg per dose was determined to be necessary to achieve consistent and significant gene silencing in tumours. At the dose of 2.5 μg, measurement of EphA2 by western blot of tumour lysate revealed superior gene-silencing effect of MePS2-1-siEphA2-DOPC compared with UM-siEphA2-DOPC (80% versus 30% reduction, respectively). We next treated mice with 2.5 μg of UM-siCon-DOPC, UM-siEphA2-DOPC, MePS2-1-siCon-DOPC and MePS2-1-siEphA2-DOPC twice weekly ( n =10). After 4 weeks of therapy, the animals were killed and necropsies were performed. UM-siEphA2-DOPC reduced the tumour burden compared with UM-siCon-DOPC group (50% reduction); however, the difference is not statistically significant. In contrast, MePS2-1-siEphA2-DOPC exhibited significant reduction in tumour weight ( Fig. 3g , 70% reduction) compared with the MePS2-1-siCon-DOPC treatment group. No group showed decreased body weight, one major indicator of toxicity ( Fig. 3h ). Overall, these results demonstrate superior gene-silencing and therapeutic effects with MePS2-1-siEphA2-DOPC compared with UM-siEphA2-DOPC. We next evaluated the pharmacokinetic profile and biodistribution pattern of MePS2-1-siEphA2-DOPC following a single i.p. injection in tumour-bearing mice. The level of siRNAs accumulated in tumours was found to be significantly higher than that observed in other major organs, including the lung, heart, liver, spleen, kidneys and brain ( Fig. 3i ). The localization of DOPC nanoliposomes to tumours was further confirmed using Cy5.5-labelled siRNAs ( Supplementary Fig. 10 ). This ability of DOPC nanoliposomes to preferentially deliver siRNAs to tumours while avoiding significant uptake in other organs is similar to that observed with several other systems, including pRNA nanoparticles [31] . The pharmacokinetic analysis of MePS2-1-siEphA2-DOPC showed an area under the curve (AUC) 0-72 of 477 pg h −1 ml −1 , clearance of 5.23 l h −1 , and volume of distribution of 26.3 l. Distribution half-life of MePS2-1-siEphA2-DOPC was 3.7 min and the elimination half-life was 9.3 h. Targeting GRAMD1B for OvCa treatment Having demonstrated that MePS2-1 siRNA has superior gene-silencing activity compared with its UM counterpart for an established target, we next assessed its silencing, and in turn, therapeutic capability for an OvCa target gene. Since acquired chemoresistance is a major contributor to patient mortality from OvCa, we sought to identify targets having substantial roles in this process. SiRNAs against approximately 22,000 individual genes were evaluated for their lethality and ability to induce taxane sensitivity in taxane-resistant epithelial OvCa cells (SKOV3-TR) ( Supplementary Data 1 ). High correlation between cell viability score was observed across triplicate plates (median coefficient of variation=8.6%), indicating high data precision in the screen. A total of 178 genes were identified to have reduced cell viability upon siRNA treatment and showed further cell death when combined with paclitaxel ( Supplementary Data 2 ). Importantly, the dose of paclitaxel used in the screen was IC 30 of that achieved in parental taxane-sensitive SKOV3ip1 cells to permit identification of genes that, when silenced, can dramatically sensitize cells to taxane treatment. Out of 178 hits, eight genes were identified to be up-regulated in OvCa epithelial cells compared to normal ovarian surface epithelial cells [32] ( Fig. 4a ). Within this group, we focused on three genes associated with the highest lethality upon knockdown when combined with paclitaxel: GRAMD1B , RBBP6 and SLC23A1 . We found that taxane-resistant OvCa cell lines (HeyA8-MDR, SKOV3-TR) showed elevated levels of GRAMD1B mRNA and protein relative to their sensitive counterparts (HeyA8, SKOV3ip1) ( Fig. 4b,c ). The expression of GRAMD1B remained unchanged for platinum resistant A2780-CP20 cells when compared with the parental line (A2780), indicating the lack of involvement of this gene in platinum resistance. GRAMD1B was also confirmed to be highly elevated in HeyA8 and SKOV3ip1 compared with the non-transformed HIO-180 ovarian epithelial cells. RBBP6 and SLC23A1 mRNA expression levels, although elevated in some OvCa lines, were not found to be increased in resistant cell lines examined ( Fig. 4b ). 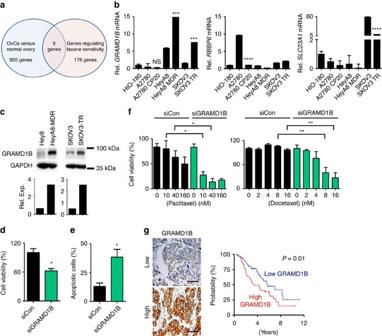Figure 4: Targeting GRAMD1B for OvCa treatment. (a) A Venn diagram for identification of novel targets for the treatment of OvCa. (b) Expression ofGRAMD1B, RBBP6andSLC23A1, in a panel of chemosensitive and chemoresistant OvCa cell lines. (c) Protein expression of GRAMD1B in taxane-sensitive (HeyA8 and SKOV3ip1) and taxane-resistant (HeyA8-MDR and SKOV3-TR) OvCa cells (n=1). Effect of GRAMD1B downregulation on (d) cell viablity and (e) apoptosis in HeyA8-MDR cells. (f) Effect of knockdown of GRAMD1B on the sensitivity of HeyA8-MDR cells to paclitaxel or docetaxel treatment. Cell viability is expressed as a percentage of that measured in siRNA monotherapy-treated wells. (g) Effect of GRAMD1B protein expression on overall survival in OvCa patients (n=156). Scale bar, 100 μm. (P-values obtained with (a–f) Student’st-test or (g) log-rank test; (b) ***P<0.001 or ****P<0.0001; compared with the corresponding chemosensitive cell line; (d–f) *P<0.05 or **P<0.01; compared with cells treated with siCon; bars and error bars represent mean values and the corresponding s.e.m.s (n=3).) Figure 4: Targeting GRAMD1B for OvCa treatment. ( a ) A Venn diagram for identification of novel targets for the treatment of OvCa. ( b ) Expression of GRAMD1B, RBBP6 and SLC23A1 , in a panel of chemosensitive and chemoresistant OvCa cell lines. ( c ) Protein expression of GRAMD1B in taxane-sensitive (HeyA8 and SKOV3ip1) and taxane-resistant (HeyA8-MDR and SKOV3-TR) OvCa cells ( n =1). Effect of GRAMD1B downregulation on ( d ) cell viablity and ( e ) apoptosis in HeyA8-MDR cells. ( f ) Effect of knockdown of GRAMD1B on the sensitivity of HeyA8-MDR cells to paclitaxel or docetaxel treatment. Cell viability is expressed as a percentage of that measured in siRNA monotherapy-treated wells. ( g ) Effect of GRAMD1B protein expression on overall survival in OvCa patients ( n =156). Scale bar, 100 μm. ( P -values obtained with ( a – f ) Student’s t -test or ( g ) log-rank test; ( b ) *** P <0.001 or **** P <0.0001; compared with the corresponding chemosensitive cell line; ( d – f ) * P <0.05 or ** P <0.01; compared with cells treated with siCon; bars and error bars represent mean values and the corresponding s.e.m.s ( n =3).) Full size image We next examined the effect of silencing GRAMD1B in the taxane-resistant cell line with the highest target expression, HeyA8-MDR ( Supplementary Data 3 , Supplementary Fig. 11 , and Fig. 4d,e ). GRAMD1B silencing via introducing siGRAMD1B into cells using Lipofectamine 2000 exhibited both lethality as monotherapy (40% decrease in cell viability and 3-fold increase in apoptosis, Fig. 4d,e ) and also taxane sensitization at 10 nM paclitaxel (>75% versus <5% cell death, siGRAMD1B plus paclitaxel versus siCon plus paclitaxel) ( Fig. 4f ). Treatment with docetaxel produced a similar pattern. Significant taxane sensitization was also observed when another GRAMD1B-targeting siRNA was transfected into cells using another transfecting reagent, Lipofectamine RNAiMax ( Supplementary Fig. 12 ). These results indicate the potential of GRAMD1B silencing in overcoming taxane resistance in OvCa. Given the preclinical efficacy after targeting GRAMD1B, we subsequently assessed the impact of tumoral GRAMD1B expression on patient survival. Immunohistochemical GRAMD1B expression was analysed against the clinical characteristics of a cohort of 156 women with mostly advanced epithelial OvCa ( Supplementary Table 2 ). High tumoral GRAMD1B expression was significantly associated with several indicators of aggressive disease, including suboptimal cytoreductive surgery (50% versus 33%, P =0.04, χ 2 test), progressive or recurrent disease (92.6% versus 74.5%, P =0.004, χ 2 test), lower median progression-free survival (0.9 versus 1.72 years, P =0.001, log-rank test) and lower overall survival (OS, 3.59 versus 6.14 years, P =0.01, log-rank test, Fig. 4g ). GRAMD1B expression remained an independent predictor of survival following multivariate analysis accounting for age, stage, grade, extent of cytoreduction and GRAMD1B expression ( P =0.02, Cox proportional-hazards model). We further investigated the relationship between tumoral GRAMD1B expression and chemotherapy response in a subset of OvCa patients ( n =32) who had suboptimal tumour debulking at the time of surgery (that is, >1 cm residual disease). Cancer antigen 125 (CA125) was used as a measure of drug response [33] . Patients who had CA125 level normalized to 35 at the end of six cycles of chemotherapy were considered responsive to treatments. It was found that 89% of patients with high tumoral GRAMD1B protein expression levels responded poorly to chemotherapy (that is, CA125>35 at the end of six cycles of chemotherapy). In contrast, patients whose tumour had low GRAMD1B expression responded significantly better to chemotherapy ( P <0.001, χ 2 test), with 91.3% of patients having normalized CA125 at the end of the therapy. Median progression-free survival was 0.61 and 2.07 years for patients with high versus low tumoral GRAMD1B expression, respectively ( Supplementary Fig. 13 ). Therapeutic effect of MePS2-1 siGRAMD1B in vitro and in vivo Having established the importance of targeting GRAMD1B in OvCa treatment, we next examined if MePS2-1 modification can significantly enhance the silencing efficiency of UM siGRAMD1B. We found that MePS2-1 siGRAMD1B efficiently silenced GRAMD1B both at the mRNA (70%, data not shown) and protein (85%) level in HeyA8-MDR cell line in the presence of serum (40 nM, Fig. 5a ). This level of GRAMD1B knockdown was significantly better than that achieved by UM siGRAMD1B (85% versus 50%). Consistent with our findings using siEphA2 and siPTMS ( Fig. 2d,e ; Fig. 3b,c ; Supplementary Fig. 5 ), MePS2-1 modification also significantly enhances the serum and intracellular stabilities of siGRAMD1B ( Supplementary Fig. 14 ) and increases its binding to Ago2 protein when compared with UM siGRAMD1B ( Fig. 5b ). Let-7a was used as a normalizing control for the Ago2 binding study as its expression is not altered by GRAMD1B silencing ( Supplementary Fig. 15 ). 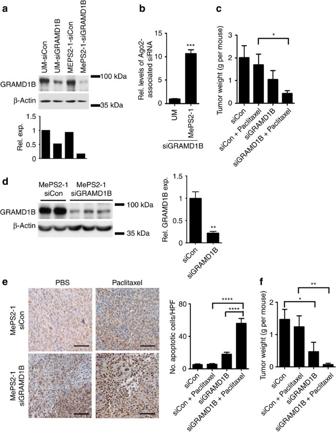Figure 5: Therapeutic effect of MePS2-1 siGRAMD1Bin vitroandin vivo. (a) Knockdown of GRAMD1B using UM and MePS2-1-modified siRNAs (40 nM, 10% FBS-containing media) (n=1). (b) Intracellular binding of UM and MePS2-1 siGRAMD1B to Ago2 in HeyA8-MDR cells (50 nM, serum-free condition). (c) Effect of MePS2-1 siGRAMD1B on tumoral response to paclitaxel treatment in HeyA8-MDR orthotopic OvCa mouse model. (d) Knockdown of GRMAD1B by MePS2-1-siGRAMD1B-DOPC in HeyA8-MDR tumours. (e) Caspase 3 activity in tumours treated with MePS2-1-siCon-DOPC or MePS2-1-siGRAMD1B-DOPC +/− paclitaxel. Scale bar, 100 μm. (f) Effect of MePS2-1 siGRAMD1B on tumoral response to paclitaxel treatment in SKOV3-TR orthotopic OvCa mouse model. (P-values obtained with Student’st-test; (b) ***P<0.001, compared with UM siGRAMD1B (n=3); (c,f) *P<0.05 or **P<0.01, compared with the corresponding control groups (n=10); (d) **P<0.01, compared with MePS2-1-siCon-DOPC group (n=2–3); (e), ****P<0.0001, compared with paclitaxel or MePS2-1-siGRAMD1B-DOPC monotherapy groups (n=10); bars and error bars represent mean values and the corresponding s.e.m. values). Figure 5: Therapeutic effect of MePS2-1 siGRAMD1B in vitro and in vivo . ( a ) Knockdown of GRAMD1B using UM and MePS2-1-modified siRNAs (40 nM, 10% FBS-containing media) ( n =1). ( b ) Intracellular binding of UM and MePS2-1 siGRAMD1B to Ago2 in HeyA8-MDR cells (50 nM, serum-free condition). ( c ) Effect of MePS2-1 siGRAMD1B on tumoral response to paclitaxel treatment in HeyA8-MDR orthotopic OvCa mouse model. ( d ) Knockdown of GRMAD1B by MePS2-1-siGRAMD1B-DOPC in HeyA8-MDR tumours. ( e ) Caspase 3 activity in tumours treated with MePS2-1-siCon-DOPC or MePS2-1-siGRAMD1B-DOPC +/− paclitaxel. Scale bar, 100 μm. ( f ) Effect of MePS2-1 siGRAMD1B on tumoral response to paclitaxel treatment in SKOV3-TR orthotopic OvCa mouse model. ( P -values obtained with Student’s t -test; ( b ) *** P <0.001, compared with UM siGRAMD1B ( n =3); ( c , f ) * P <0.05 or ** P <0.01, compared with the corresponding control groups ( n =10); ( d ) ** P <0.01, compared with MePS2-1-siCon-DOPC group ( n =2–3); ( e ), **** P <0.0001, compared with paclitaxel or MePS2-1-siGRAMD1B-DOPC monotherapy groups ( n =10); bars and error bars represent mean values and the corresponding s.e.m. values). Full size image Moving into an orthotopic mouse model, we injected HeyA8-MDR cells into the peritoneal cavity and, after 1 week, mice were divided into four treatment groups: (a) MePS2-1-siCon-DOPC, (b) MePS2-1-siGRAMD1B-DOPC, (c) MePS2-1-siCon-DOPC plus paclitaxel or (d) MePS2-1-siGRAMD1B-DOPC plus paclitaxel. Dosing was twice weekly for siRNA and weekly for paclitaxel (at a sub-therapeutic 100 μg dose), followed by tumour excision and quantification after 5 weeks of treatment. No significant reduction in tumour burden was observed for sub-therapeutic paclitaxel with MePS2-1-siCon-DOPC treatment group, as expected ( Fig. 5c ). However, MePS2-1-siGRAMD1B-DOPC alone resulted in 50% reduction in tumour burden, consistent with our in vitro findings ( Fig. 4d ). Combining it with paclitaxel induced a 55% further reduction in total tumour weight compared with MePS2-1-siGRAMD1B-DOPC monotherapy, indicating the potential for taxane sensitization after GRAMD1B silencing. The reduction of GRAMD1B levels in tumours by MePS2-1-siGRAMD1B-DOPC was significant, with the protein level being downregulated by 80% in tumours from mice treated with MePS2-1-siGRAMD1B-DOPC ( Fig. 5d ). This downregulation of GRAMD1B in tumours was also significantly associated with the induction of cleaved caspase 3 ( Fig. 5e ). This is consistent with the increased level of apoptotic cells observed following GRAMD1B silencing in vitro ( Fig. 4e ). Replicating the experiment with a different GRAMD1B-targeted siRNA sequence in SKOV3-TR, another taxane-resistant OvCa model, produced a similar therapeutic effect ( Fig. 5f ). In this model, mice treated with both MePS2-1-siGRAMD1B-DOPC and paclitaxel had an 80% further decrease in tumour burden compared with mice treated with MePS2-1-siGRAMD1B-DOPC alone, which again indicated the role of GRAMD1B in taxane resistance. Importantly, in both of the models tested, there was no alteration in mouse body weights in any of the treatment groups ( Supplementary Fig. 16 ). Recent advances in high-throughput genomic and computational tools have facilitated the identification of new targets with translational potential [34] . Combining novel MePS2 siRNA chemistry with a whole-genome lethality screen aimed at identifying novel genes involved in taxane resistance, we demonstrate, for the first time, the feasibility of using highly potent MePS2-modified siRNAs for effective therapeutic targeting. We show that GRAMD1B, a gene identified through our high-throughput screening and analyses, has both high biological and clinical importance. Using it as a model system, we demonstrate that robust gene silencing in tumours can be achieved following systemic administration of MePS2-modified siRNAs. This ultimately led to significant re-sensitization of chemoresistant ovarian tumours to taxane therapy. Most of the chemical modification strategies, to date, have focused on improving siRNA stability in serum [7] . While this is critical, improving siRNA potency at target sites following systemic administration still remains the major obstacle to clinical translation of siRNAs [5] , [6] . Through a systematic approach, we have identified a unique combination of 2′-OMe and PS2 that significantly improves stability and potency of siRNAs simultaneously ( Fig. 6 ). We first confirmed that the increase in potency could not be explained by the design’s enhanced stability, consistent with previous findings that this mechanism has a limited role within rapidly dividing cells [35] , and then investigated other potential causes. 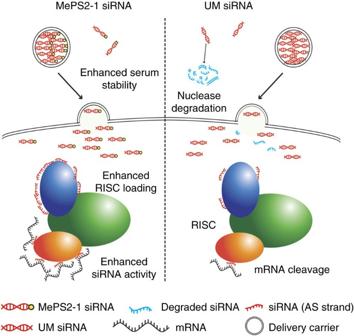Figure 6: A schematic representation of mechanisms by which MePS2 modification enhances siRNA activity. MePS2-1 modification enhances serum stabilty of siRNAs and promotes the loading of the antisense strand into RISC. Figure 6: A schematic representation of mechanisms by which MePS2 modification enhances siRNA activity. MePS2-1 modification enhances serum stabilty of siRNAs and promotes the loading of the antisense strand into RISC. Full size image We discovered that MePS2 modification further enhances the loading of siRNAs to RISC, compared with PS2 modification, resulting in enhanced silencing. While the addition of methyl groups typically elevates Tm , we show here that the addition of 2′-OMe to PS2-modified siRNAs does not increase the Tm of the siRNA duplex, suggesting a unique property arising from this combination. The computational modelling also indicates an unusual favourable stereoelectronic effect on the siRNA backbone following MePS2 modification. These results indicate that MePS2 modification can improve the interaction of siRNA with RISC via several mechanisms, namely the thiol–protein interaction [26] , [27] , [36] , modulation of Tm and altered stereoelectronics. This is in contrast to currently existing modifications, where RISC loading efficiency is dependent on alteration in Tm , thus leading to variable silencing effects depending on the Tm of the sequences to be modified [20] , [37] . Hence, MePS2 modification has a unique potential to provide more consistent, sequence-independent, silencing effects compared with existing chemistries. In summary, we show that 2′-OMe and PS2 combination not only significantly increases the serum stability of siRNAs but also triggers a more potent intrinsic RNAi response than the individual modifications. In addition to its achiral nature that favors clinical translation, we have demonstrated the ability of MePS2 modification to overcome major obstacles of bringing siRNA therapeutics into the clinic. It is anticipated that further understanding the unique and advantageous interaction between 2′-OMe and PS2 moieties will facilitate the rational design of highly potent and stable siRNAs in the near future. Cell lines The OvCa cell lines, SKOV3ip1 and HeyA8, were obtained from ATCC and were maintained in RPMI 1,640 supplemented with 15% FBS and 0.1% gentamicin sulphate (Gemini Bioproducts; Calabasas, CA) [38] . SKOV3-TR and HeyA8-MDR were kind gifts from Dr Isaiah Fidler, Department of Cancer Biology, University of Texas MD Anderson Cancer Centre and Dr Michael Seiden, Department of Medicine, Massachusetts General Hospital, respectively. SiRNA synthesis SiRNAs were synthesized at AM Biotechnologies. All sequences are listed in Supplementary Table 3 . Modified and UM 21-nt RNAs (sense and antisense strands) were synthesized on the 1 μmol scale on an Expedite 8909 DNA/RNA Synthesizer using commercial available 5′-DMT-2′- O -TBDMS nucleoside (A Bz , C Ac , G Ac and U) phosphoramidite monomers and 5′-DMT-2′-OMe nucleoside (A Bz , C Ac , G Ac and U) phosphoramidite monomers as well as in house produced 5′-DMT-2′-OMe nucleoside (A Bz , C Ac , G Ac and U) thiophosphoramidite monomers [15] , [16] , [28] . All oligonucleotides were synthesized in DMT-off mode. After completion of the synthesis, the solid support was suspended in ammonium hydroxide/methylamine (AMA) solution (prepared by mixing 1 volume of ammonium hydroxide (28%) with 1 volume of 40% aqueous methylamine) and heated at 65 °C for 15 min to release the product from the support and to complete the removal of all protecting groups except the TBDMS group at the 2′ position. The solid support was filtered, and the filtrate was concentrated to dryness. The obtained residue was resuspended in 115 μl of anhydrous DMF and then heated for 5 min at 65 °C to dissolve the crude product. Triethyl amine (60 μl) was added to each solution, and the solutions were mixed gently. Triethyl amine·3HF (75 μl) was added to each solution, and the tubes were then sealed tightly and incubated at 65 °C for 2.5 h. The reaction was quenched with 1.75 ml of DEPC-treated water. Purification was performed on an Amersham Biosciences P920 FPLC instrument fitted with a Mono Q 10/100 GL column [39] . The structures of the modified RNAs were confirmed by ESI-MS and 31P-NMR. The assembly of the resulting duplexes was confirmed on a 4% agarose gel electrophoresis. For in vivo experiments, ammonium counter cation was replaced by sodium cation. In vitro siRNA transfection and luciferase assays Cells were transfected with 10–100 nmol l −1 of specified siRNAs using Lipofectamine 2000 or Lipofectamine RNAiMax reagent (Invitrogen) at 3 μl reagent: 1 μg siRNA ratio [21] . Cells were treated with siRNAs for 4 h in serum-free or 10% FBS-containing media before incubation in fresh complete media for the specified timeframe. GoClone pLightSwitch luciferase reporter constructs containing AS and S siRNA target sequences were obtained from SwitchGear genomics (Menlo Park, CA). AS construct contains the following sequence: 5′-CAAAGGGTGGGACCTGATGCAGAACATCA TGAATGACATGCCGATCTACATGTACTCCGTGTGCAACGTGATGTCTGGCGAC-3′. S construct contains the following sequence: 5′-ACCTGATGCAGAACATCATGAACAT GTAGATCGGCATGTCATACTCCGTGTGCAACGTGATGTCT-3′. SKOV3ip1 cells were transfected with FuGENE HD reagent in a 96-well plate with specified siRNAs (100 nM) along with S or AS reporter construct, and Cypridina TK control construct (pTK-Cluc) [40] . After 24 h of transfection, luciferase activity was obtained using LightSwitch Dual Luciferase assay kits. Luciferase activity was normalized with the Cypridina TK control construct. All assays were performed in triplicate. Quantitative reverse transcription PCR RNA was isolated from cells, Ago2 pulldown products, blood samples and tissues using Trizol (Invitrogen) according to the manufacturer’s protocol. Using 1 μg of RNA, cDNA was synthesized by using a Verso cDNA kit (Thermo Scientific) as per the manufacturer’s instructions. Analysis of mRNA levels was performed on a 7500 Fast Real-Time PCR System (Applied Biosystems) with SYBR Green-based qRT–PCR. PCR was performed with reverse-transcribed RNA and 100 ng μl −1 of forward and reverse primers in a total volume of 20 μl (ref. 38 ). All primer sequences for mRNA detection are listed in Supplementary Table 4 . Each cycle consisted of 15 s of denaturation at 95 °C and 1 min of annealing and extension at 60 °C (40 cycles). Stemloop PCRs for siRNA detection were performed using TaqMan miRNA assays followed by SYBR Green-based qRT–PCR [41] . Stemloop primers used to synthesize cDNA are listed in Supplementary Table 5 . Respective forward primers as well as a common reverse primer used for qRT–PCR are listed in Supplementary Table 4 . For miRNA quantification, total RNA was isolated using Trizol (Invitrogen) extraction. TaqMan miRNA assays (Applied Biosystems) were used for reverse transcription and qRT–PCR was performed according to the manufacturer’s instructions. For microRNA detection, Ambion assay probe sets were used according to the manufacturer’s protocol. The relative amount of mRNA/siRNA in each sample was normalized to β-actin mRNA, RNU44, RNU6B or respective miRNAs. Melting profiles of siRNAs Complementary RNA strands were mixed in 10 mM Tris-HCl buffer (pH 7.4) with 100 mM NaCl, and 0.1 mM ethylenediaminetetraacetic acid (EDTA) at a final concentration of 2 μM. Annealing was performed at a temperature gradient of 1.5 °C min −1 , from 85 to 15 °C. Melting profiles were measured using a temperature gradient of 1 °C min −1 , from 15 to 85 °C, with the detector set at 260 nm ( n =3–6). CD measurements CD spectra were recorded on a CD6 dichrograph (Jabin-Yvon) using cells with 0.5 cm path length, 2 nm bandwidth and 1–2 s integration time. Each spectrum was smoothed with a 25-point algorithm. The spectra from 200–340 nm were recorded at 25 °C in the same buffer as in the melting experiments ( n =3). The concentration of the two complementary RNA oligonucleotides was ca . 2 μM. Western blot Protein lysates were prepared from cultured cells or tumours using modified RIPA buffer (50 mM Tris-HCl (pH 7.4), 150 mM NaCl, 1% Triton, 0.5% deoxycholate) plus 25 μg ml −1 leupeptin, 10 μg ml −1 aprotinin, 2 mM EDTA and 1 mM sodium orthovanadate [38] . Membranes were probed with primary antibodies against EphA2 (1:1,000, Millipore, 05-480), β-actin (1:5,000, Sigma, A5316), vinculin (1:2,500, Sigma, V9131), GAPDH (1:5000, Sigma, G8795), Ago2 (1:100, Wako Chemicals, 015-22031) and GRAMD1B (1:500, Sigma, HPA008557) in 5% skim milk in TBS-T. Quantification was performed using ImageJ. Full scans of important western blots are provided in Supplementary Fig. 17 . Intracellular Ago2-binding study Cells were lysed at 7 h post transfection using ice-cold lysis buffer (50 mM Tris-HCl at pH 7.5, 200 mM NaCl, 0.5% Triton, 2 mM EDTA, 1 mg ml −1 heparin and protease inhibitor cocktail) [42] , [43] . Ago2 antibody (Wako Chemicals, 015-22031, 20 μl) was absorbed onto magnetic protein G Dynabeads (Invitrogen, 40 μl) by incubation at 4 °C for 2 h on a rotator. The beads were then washed twice with lysis buffer to remove unbound antibodies. Following washing, beads were incubated with protein lysate (360 μg) overnight at 4 °C on a rotator. Following removal of unbound proteins, bound material was eluted from beads using 50 μl of 0.1 M glycine (pH 2.3) for 15 min at RT. Eluted fractions were neutralized immediately with an equal volume of 1 M Tris-HCl (pH 8) and then treated with 20 U of proteinase K for 10 min at 65 °C (ref. 44 ). The amount of Ago2-bound siRNA was then quantified using stemloop PCR technique. For the biotin-siRNA pulldown experiment, strepavidin beads were blocked and incubated with cell lysates at 4 °C for 2 h (ref. 42 ). The amount of siRNA-associated Ago2 was quantified via western blotting. Serum stability assay SiRNAs (1.33 μg) were incubated in 10 μl of 10% FBS in PBS at 37 °C for up to 24 h. All samples were separated in 20% polyacrylamide gels. The percentage of intact siRNA present was quantified using ImageJ. Immunogenicity of siRNAs Bone marrow progenitor cells were isolated from C57BL/6 mice and were differentiated into dendritic cells in vitro for 7 days using FLT3 ligand (100 ng ml −1 ; PeproTech). Cells were treated with 75 nM of siRNAs for 6 h in serum-free media using RNAiMax. A high interferon-inducing siRNA sequence (BP1Mod2; Supplementary Table 3 ) and CpG 2216 (1 μg ml −1 , Sigma) were used as positive controls. The level of IFN-α and TNF-α in the culturing media was assessed using murine IFN-α and TNF-α ELISA kits at 2, 6 and 24 h following transfection (R&D Systems). For TLR7 experiments, peripheral blood mononuclear cells were obtained from wild-type and TLR7-KO C57BL/6 mice and were treated with 75 nM of siRNAs for 6 h. IFN-α and TNF-α levels in the culturing media was measured 24 h post transfection. For in vivo studies, serum was collected from mice at 2, 6 and 24 h post siRNA treatment and IFN-α and TNF-α levels were measured as described above. Liposomal nanoparticle preparation SiRNAs for in vivo delivery were incorporated into DOPC liposomes [21] . DOPC and siRNA were mixed in the presence of excess tertiary butanol at a ratio of 1:10 ( w / w ) siRNA/DOPC. Tween 20 was added to the mixture in a ratio of 1:19 Tween 20:siRNA/DOPC. The mixture was vortexed, frozen in an acetone/dry ice bath and lyophilized. Before in vivo administration, this preparation was hydrated with PBS. Orthotopic in vivo models of OvCa Female athymic nude mice (8–12 weeks old) were obtained from the National Cancer Institute, Frederick Cancer Research and Development Center (Frederick, MD). All mouse studies were approved and supervised by the MD Anderson Cancer Center Institutional Animal Care and Use Committee. For therapeutic experiments, 10 mice were assigned per treatment group. This sample size gave 80% power to detect a 50% reduction in tumour weight with 95% confidence. To establish intraperitoneal tumours, cells were injected into the peritoneal cavity i.p. at a concentration of 5 × 10 6 cells per ml (200 μl per injection). All mice were treated with siRNAs (2.5 or 5 μg for EphA2 and GRAMD1B experiments, respectively) twice weekly beginning at 1 week following tumour cell injection. Paclitaxel (100 μg) was injected i.p. once weekly. Mice ( n =10 per group) were monitored for adverse effects and tumours were harvested after 5 weeks of therapy or when any of the mice began to appear moribund. Mouse weight, tumour weight and the number/location of tumour nodules were recorded. Tumour tissues were fixed in formalin for paraffin embedding or was snap frozen for lysate preparation [21] . For gene silencing (1.25 and 2.5 μg), immune toxicity (5 μg), pharmacokinetic (2.5 μg) and biodistribution studies (2.5 μg), single dose of siRNA was administered i.p. once tumours became palpable. Blood and/or tissues samples were collected at specified time points for RNA/protein extraction or ELISA assay. For the fluorescence-based biodistribution study, Cy5.5-labelled siRNAs were administered i.p. and 48 h later, fluorescence imaging of excised tumour and organs was performed using the Xenogen IVIS 200 system [40] . Cy5.5 fluorophore excitation (678 nm) and emission (703 nm) filters were used. Using Living image 2.5 software, regions of interest were drawn for each organ and the total radiant efficiency ps −1 μW −1 cm 2 was measured. Pharmacokinetic analysis Blood concentrations of siRNA at the indicated times, C ( t ), were expressed as pg siRNA per ml of blood. Pharmacokinetic parameters were determined by fitting the C ( t ) with a two-compartment model using the MULTI programme [45] . The AUC of the blood concentration time was calculated by integration of C ( t ) up to 72 h following administration. Volume of distribution was calculated by dividing the injected dose by C(0). CL total was calculated by dividing injected dose by AUC. Microarray and pathway enrichment analysis HeyA8-MDR cells were treated with siGRAMD1B and total RNA was extracted 48 h following transfection using mirVana RNA isolation labelling kit (Ambion). Five hundred nanograms of total RNA were used for labelling and hybridization on a Human HT-12 v4 Beadchip (Illumina) according to the manufacturer’s protocols [46] . After the bead chips were scanned with an Illumina BeadArray Reader (Illumina), the microarray data were normalized using the quantile normalization method in the Linear Models for Microarray Data (LIMMA) package in the R language environment. The expression level of each gene was transformed into a log2 base before further analysis. GEOID for the microarray data is GSE54459. The top 10 pathways perturbed by siGRAMD1B treatment were identified using NetWalker software [47] . Each interaction in the global network of biological relationships was scored based on combined assessment of the network connectivity and the input data. Biological pathways were ranked based on geometric P- values. SiRNA lethality screen SKOV3-TR cells used for the screen were maintained in antibiotic-free RPMI1640 supplemented with 10% FBS [48] and were authenticated prior to their utilization in the screen. For the screen, SKOV3-TR (2,000 cells per well) were transfected using siRNAs in individual wells of black 384-well plates for 48 h. Transfection was performed using a pool of four individual siRNAs targeting individual genes (siGenome Smart pool, G-004605, Dharmacon) using Dharmafect 1 (Dharmacon) [49] . SiTOX was used as a control for transfection efficiency. Non-targeting siRNA number 4 (siOTP4, Dharmacon) was used as a transfection control in all experiments. In summary, 0.2 μl of 20 μM siRNA was mixed with 0.2 μl of Dharmafect 1 and 20 μl of Optimem medium (Invitrogen) for 20 min in a well of 384-well plate and overlaid with 80 μl of cell suspension (2,000 cells) in antibiotic-free RPMI1640 supplemented with 10% FBS. This gave a final siRNA concentration of 40 nM per well. For each plate, four types of control were included: siOTP4 as a negative control (16 wells), siTOX as a control for transfection efficiency (8 wells), cells only (24 wells) and blank wells (16 wells). Following siRNA treatment, cells were treated with paclitaxel (3.5 nM). All experiments were performed at 37 °C in the presence of 5% CO 2 . Finally, cell viability was determined using 3-(4,5-dimethylthiazol-2-yl)-2,5-diphenyltetrazolium bromide (MTT, USB Corporation) as per manufacturer’s instruction 3 days after treatment and signal was detected using a PHERAstar FS plate reader (BMG Labtech). Following data collection, the values in each plate were centered on 100 using median scaling [49] and cell viabilities were expressed as percentages of siOTP4-treated samples. Student’s t -test was used to examine chemosensitization following conversion of raw values to log2 scale. Immunohistochemistry analysis Staining was performed in paraffin-embedded tumour sections [21] . For patient samples, tissue microarray slides containing 156 OvCa samples were obtained from MD Anderson Cancer Center following approval by the Institutional Review Board. Antigen retrieval was performed using citrate buffer (pH 6) or Borg Decloaker solution (Biocare Medical, BD1000 S-250) for GRAMD1B and cleaved caspase 3, respectively. Slides were incubated with primary antibodies against GRAMD1B (1:100 dilution, Sigma, HPA008557) or cleaved caspase 3 (1:200, BioCare Medical, CP229A) overnight, followed by incubation with horseradish peroxidase-conjugated or biotinylated/streptavidin anti-Rabbit secondary antibodies, respectively (Jackson Laboratory, 111-036-047 and BioCare Medical, GR602 H). The stained slides were scored by two investigators blinded to the treatment groups or patient survival information. For in vivo samples, 5–10 random fields at × 200 magnification for each tumour were examined. For patient samples, a scoring system, which considered both the intensity of staining and the percentage of cells stained, was used [46] , [50] . H scores of >100 and ⩽ 100 were defined as high and low expression, respectively. Cell viability assays HeyA8-MDR cells were transfected with siRNAs (100 nM) on day 1 and 3 before paclitaxel or docetaxel treatment. Cell viability was assessed 3 days following taxane treatment using MTT assay as per manufacturer’s protocol. Statistical analysis Kaplan–Meier plots were constructed and a log-rank test was used to determine differences among survival curves according to tumoral GRAMD1B expression level [46] , [50] . Contingency tables and Fisher's exact test or χ 2 test were used to evaluate the relationship between death and categorical variables. Multivariate analyses were performed with the use of a Cox proportional-hazards model to examine the effects of tumoral GRAMD1B expression on death from disease while adjusting for other covariates. χ 2 test was performed to assess the effect of tumoral GRAMD1B expression on drug response. For siRNA lethality screen, Student’s t -test was used to examine chemosensitization following conversion of raw values to log2 scale. For other assays, Student’s t -test was performed to examine the difference between control and treatment groups. Apoptosis assay Apoptosis was studied using the Annexin V apoptosis detection kit (BD Biosciences) according to the manufacturer's protocol [38] . Apoptotic cells were analysed using a FACSCalibur flow cytometer (BD Biosciences). CellQuest Pro software (BD Biosciences) was used to determine the number of apoptotic cells. Modelling of siRNA:PAZ domain interactions Coordinates of the complex between a 9 mer siRNA and the PAZ domain from human Argonaute eIF2c1 were retrieved from the Protein Data Bank ( http://www.rcsb.org ; PDB ID code 1si2 (ref. 29 )). The programme UCSF Chimera [51] was used to convert the sequence of the last four nucleotides in the siRNA from the 1si2 crystal structure to match the sequence and chemistry of MePS2-1 (...ACUdCdU-3′ and …AU MeS2 G MeS2 dTdT-3′, respectively). Changes to reflect the chemistries of the Me-1 and PS2-1 siRNAs were accomplished in a similar manner. Side chain torsion angles of C270 and M273 were adapted in USCF Chimera, and the programme was used for measuring distances and producing figures. The complex models generated were not subjected to energy minimization with either molecular mechanics or dynamic approaches. The important role of M273 in stabilizing the siRNA–PAZ interaction is reflected by the change in K d upon mutation of residue 273 from methionine to alanine [29] . The side chain of M273 snakes along the terminal base pair of the siRNA duplex, and the mutation to alanine abolishes this stacking interaction and doubles the K d . The effect of hydrophobic interactions between siRNAs and M273/C270 on K d was also examined. How to cite this article : Wu, S. Y. et al . 2′-OMe-phosphorodithioate-modified siRNAs show increased loading into the RISC complex and enhanced anti-tumour activity. Nat. Commun. 5:3459 doi: 10.1038/ncomms4459 (2014). Accession codes : The microarray data have been deposited in the Gene Expression Omnibus database under accession code GSE54459 .